Coupled nitrification and N2gas production as a cryptic process in oxic riverbeds The coupling between nitrification and N 2 gas production to recycle ammonia back to the atmosphere is a key step in the nitrogen cycle that has been researched widely. An assumption for such research is that the products of nitrification (nitrite or nitrate) mix freely in the environment before reduction to N 2 gas. Here we show, in oxic riverbeds, that the pattern of N 2 gas production from ammonia deviates by ~3- to 16-fold from that predicted for denitrification or anammox involving nitrite or nitrate as free porewater intermediates. Rather, the patterns match that for a coupling through a cryptic pool, isolated from the porewater. A cryptic pool challenges our understanding of a key step in the nitrogen cycle and masks our ability to distinguish between sources of N 2 gas that 20 years’ research has sought to identify. Our reasoning suggests a new pathway or a new type of coupling between known pathways in the nitrogen cycle. Nitrogen is a key bio-element for life on Earth, integral to proteins and the very DNA that tells life what to do. A vast reservoir of nitrogen resides in the atmosphere as N 2 gas, unavailable to the majority of life until being fixed by either biological or anthropogenic nitrogen fixation. Life’s organically-bound nitrogen in turn decays to ammonia following excretion or death. To complete the cycle, first nitrogen must be oxidised to nitrite or nitrate which can then be reduced back to atmospheric N 2 gas. This process of ammonia oxidation—known as nitrification—typically occurs in two stages carried out by specialised aerobic chemoautotrophic ammonia- and nitrite-oxidising microbes, for example, in soils, sediments, freshwater, or marine ecosystems (Eqs. 1 and 2 , respectively): 
    2NH_4^ + + 3O_2 → 2NO_2^ - + 2H_2O + 4H^ +     Δ G^∘' = - 270 kJ ( per NH_4^ + )
 (1) 
    2NO_2^ - + O_2 → 2NO_3^ -                 Δ G^∘' = - 79 kJ (per NO_2^- )
 (2) Nitrite and nitrate can then be reduced to N 2 gas either alone, in a phylogenetically widespread form of microbial anaerobic respiration termed denitrification [1] (Eq. 3 a, b) or, in combination with ammonia, in a phylogenetically narrow respiratory pathway termed anaerobic ammonia oxidation, namely anammox [2] (Eq. 4 ). 2NO_3^ - + 10e^ - + 12H^ + →N_2 + 6H_2O    Δ G^∘' = - 360 kJ (per NO_3^ - )
 (3a) 
    2NO_2^ - + 6e^ - + 8H^ + →N_2 + 4H_2O      Δ G^∘' = - 282 kJ (per NO_2^ - )
 (3b) 
    NH_4^ + + NO_2^ - →N_2 + 2H_2O          Δ G^∘' = - 358 kJ
 (4) In addition, smaller amounts of N can be returned to the atmosphere as nitrous oxide (N 2 O) but we do not consider those further here [3] , [4] , [5] . Combinations of Eqs. ( 1 ) to ( 4 ) recycle ammonia back into atmospheric N 2 gas and this coupling between aerobic nitrification and anaerobic N 2 gas production is a key concept in the nitrogen cycle, controlling ecosystem production and the abundance of life on Earth [6] , [7] . Besides the now accepted reactions described in Eqs. ( 1 ) to ( 4 ), Broda’s original thermodynamic predictions that drove the quest for anammox [8] , [9] also included the potential for complete aerobic ammonia oxidation to N 2 gas—that, to the best of our knowledge—has yet to be observed in nature: 
    4NH_4^ + + 3O_2 → 2N_2 + 6H_2O + 4H^ +       Δ G^∘' = - 316 kJ (per NH_4^ + )
 (5) In estuarine or coastal sea sediments, combinations of recognised aerobic and anaerobic metabolisms (Eqs. 1 to 4 ) buffer the flux of terrestrial nitrogen out to sea and are considered to be physically divided between the oxic and anoxic sediment layers—albeit by only a few tenths of millimetres [10] . In rivers, nitrite and nitrate borne from aerobic nitrification (Eqs. 1 and 2 ), in either the surrounding catchment soils or the riverbed itself, can be transported over large distances (1–100 km) before some 47 Tg N per year is removed from the fluvial network as N 2 gas [11] , [12] , [13] . Regardless of the setting, the important point to appreciate here is that the products of aerobic nitrification (e.g., nitrate and nitrite) are assumed to be free to mix with any existing nitrate and nitrite in the surrounding porewater before they are subsequently metabolised, anaerobically, to N 2 gas. That is, there is—in effect—only one pool of nitrate and nitrite awaiting reduction to N 2 gas regardless of their origins. Indeed, this concept of free mixing between substrates lies at the very heart of the common 15 N isotope pairing techniques used to disentangle and quantify the cycling of nitrogen in sediments that are major sources of N 2 gas on Earth [11] , [14] , [15] . Most research into the coupling between aerobic nitrification and anaerobic N 2 gas production in sediments has studied the two separately using either oxic or anoxic incubations, respectively [16] , but now work including oxygen is increasing [17] . Previously we demonstrated [18] that oxic (~30% to 100% of air-saturation for oxygen) gravel and sandy riverbed sediments harbour a coupling between aerobic nitrification and, seemingly, anaerobic N 2 gas production with that production being attributed to a combination of denitrification and anammox [18] . We now show that the pattern of N 2 gas production from ammonia in these oxic riverbeds violates the prevailing concept that coupled nitrification and N 2 gas production is a two-step process with free nitrite or nitrate as intermediates. Not only does this challenge our understanding of a key coupling in the nitrogen cycle but it also masks our ability to distinguish between denitrification and anammox as sources of N 2 gas. Indeed, it may actually suggest a new pathway or at least a new type of coupling between known pathways in the nitrogen cycle. N 2 gas production is independent from porewater nitrite or nitrate Following on from our original work [18] on nitrification and putative anaerobic N 2 gas production in oxic riverbeds, we wanted to explore further how these two processes are coupled. 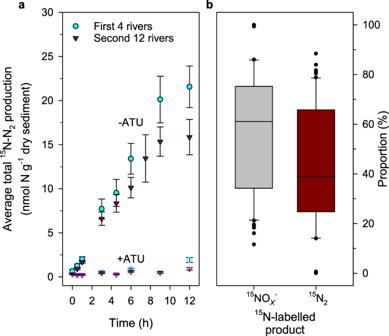Fig. 1: Oxic incubations with15N-ammonia tracer produce both15N2gas and15NOx−. aOverall average production of total15N-N2(i.e.,29N2and30N2) over time in the presence or absence of the inhibitor of ammonia mono-oxygenase, allylthiourea (ATU). The first 4 rivers (cyan circles,n= 40, 4 rivers x 5 replicates x 2 treatments at each time point, ± 1 s.e.) and the follow-up across 12 rivers (purple triangles,n= 60, 12 rivers x 5 replicates at each time point, ± 1 s.e.); open coloured symbols are the same plus ATU (see Table1).bProportions of oxidised15N-ammonia tracer froma, recovered as either15NOx−or15N2across the 12 rivers (n= 60 as fora). Upper and lower box boundaries are 75thand 25thpercentiles, respectively, upper and lower whiskers are 90thand 10thpercentiles, respectively, the extreme outliers the maxima and minima and the horizontal line the centre, median value. We began by collecting sediment from four rivers—two each of predominantly gravel and sand and then extended our sampling to a total of twelve rivers (Supplementary Figure 1 and Supplementary Table 1 ). We added 15 N-ammonia to oxic sediment microcosms (see Methods) to trace the coupling between nitrification and N 2 gas production both with and without the inhibitor of aerobic nitrification, allylthiourea [19] (~80 µM ATU in the porewater, Treatments 1 & 2, Table 1 and Methods) that does not inhibit denitrification or anammox [2] , [20] . As before [18] , we measured the immediate production of 15 N-N 2 -gas that was stopped by inhibiting the first step (Eq. 1 ) of aerobic 15 N-ammonia oxidation with ATU (Fig. 1a , Table 1 ). The coupling between aerobic ammonia oxidation and N 2 gas production was clearly strong, however it was not complete. For example, across the twelve rivers, approximately 60% (Fig. 1b ) of the oxidised 15 N-ammonia tracer was recovered from the porewater as 15 NO x − , i.e., as either 15 N-nitrite (Eq. 1 ) or the final product of nitrification, 15 N-nitrate (Eq. 2 ) e.g., 15 NO x − is the sum of 15 NO 2 − and 15 NO 3 − . Table 1 Summary of total 15 N-N 2 production in oxic incubations with 15 NH 4 + or 15 NO 2 − . Mixed-effects models were used to estimate overall rates of total 15 N-N 2 production for the incubations in Fig. 1a . Treatments 1 to 6 were applied to sediments from the first set of 4 rivers, and then just treatments 1 and 2 for the subsequent set of 12 rivers. Model fitting was carried out in the lme4 package in R [45] and rate estimates, standard errors (s.e.) and 95% confidence intervals derived using emtrends from the emmeans package (see Methods). Significant production ( bold ) of 15 N-N 2 was only measured with treatments 1 and 3. Full size table Fig. 1: Oxic incubations with 15 N-ammonia tracer produce both 15 N 2 gas and 15 NO x − . a Overall average production of total 15 N-N 2 (i.e., 29 N 2 and 30 N 2 ) over time in the presence or absence of the inhibitor of ammonia mono-oxygenase, allylthiourea (ATU). The first 4 rivers (cyan circles, n = 40, 4 rivers x 5 replicates x 2 treatments at each time point, ± 1 s.e.) and the follow-up across 12 rivers (purple triangles, n = 60, 12 rivers x 5 replicates at each time point, ± 1 s.e. ); open coloured symbols are the same plus ATU (see Table 1 ). b Proportions of oxidised 15 N-ammonia tracer from a , recovered as either 15 NO x − or 15 N 2 across the 12 rivers ( n = 60 as for a ). Upper and lower box boundaries are 75 th and 25 th percentiles, respectively, upper and lower whiskers are 90 th and 10 th percentiles, respectively, the extreme outliers the maxima and minima and the horizontal line the centre, median value. Full size image The presence of 15 N-ammonia and 15 N-NO x − together in the porewater generates two 15 N-labelled substrate pools. The fraction of the pool labelled with 15 N is termed F A for ammonia (NH 3 ) and F N for NO x − (Eqs. 10 and 11 in Methods). Theoretically, combinations of Eqs. ( 1 ) to ( 4 ) can draw on these two substrate pools ( F A and F N ) to produce both the single- 15 N-labelled, 29 N 2 gas (e.g., 14 N, 15 N) and the double- 15 N-labelled, 30 N 2 gas (e.g., 15 N, 15 N) which we illustrate schematically in Fig. 2a . Note that denitrification can draw on NO x − as either NO 2 − or NO 3 − but anammox is solely fuelled by NO 2 − . The published and accepted mathematical framework [21] (See derivation of equations in Supplementary Note 1 ) tells us that the fraction of 15 N-labelling in each of the substrate pools ( F A and F N ) must influence the ratio of 29 N 2 to 30 N 2 (here termed R ) and the overall fraction of 15 N in the N 2 gas produced e.g., the overall blend of 28 N 2 , 29 N 2 and 30 N 2 (here termed F N 2 ) [21] , [22] . While complex, the accepted framework also tells us that so long as we know what fraction of each component part ( F A , F N and F N 2 ) is labelled with 15 N, then we can still calculate how the N 2 gas is produced e.g., by anammox or denitrification and understand the nature of this key coupling in the nitrogen cycle [21] , [22] . Fig. 2: Accepted and proposed cryptic couplings in oxic N cycling. a 15 NH 4 + tracer is added to oxic sediments to mix with 14 NH 4 + in the porewater, with the fraction of 15 N labelling known as F A . Through reactions 1 and 2, 14 NH 4 + and 15 NH 4 + are oxidised aerobically to 14,15 NO 2 − and 14,15 NO 3 − to generate a 14,15 NO x − pool with 15 N labelling known as F N . NO 3 − and/or NO 2 − can be denitrified to N 2 gas (reactions 3a, 3b), or NO 2 − can oxidise NH 4 + anaerobically through anammox to N 2 gas (reaction 4). Regardless of the precise setting and combination of reactions, all substrates and products are free to mix and the measured ratio of 29 N 2 to 30 N 2 produced ( R ) can be predicted from the measured 15 N labelling in the porewater. The downwards pointing orange arrow indicates NO 3 − respiration to NO 2 − that we do not consider further here. b In contrast, our measured values for R cannot be predicted using the measured fraction of 15 N labelling in the porewater ( F A and F N ) and known combinations of reactions 1 to 4 but can only be approximated assuming a cryptic element ( F N cry ). A cryptic element could be a hidden substrate pool (6, novel or known) or novel parts of existing processes (7, e.g., complete nitrifier-denitrification beyond N 2 O to N 2 ) and/or a completely new pathway (reaction 5 e.g., complete aerobic ammonia oxidation to N 2 ) or cryptic combinations of known pathways after partial aerobic ammonia oxidation to nitrite (reactions, 1, 3b, 4). Full size image We tested the validity of this accepted mathematical framework by changing the fraction of porewater NO x − labelled with 15 N ( F N ) and looking for how this influenced the ratio of 29 N 2 to 30 N 2 produced ( R ). First we directly decreased F N by adding 14 N-nitrite to dilute the 15 N-nitrite accumulating in the porewater from the oxidation of 15 N-ammonia (Treatments 3 and 4, Table 1 ). Surprisingly, diluting F N had no discernible effect on the values for R produced in the two sets of incubations (Fig. 3b . 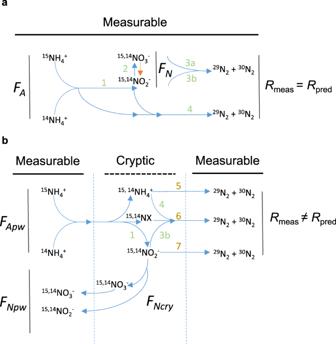Fig. 2: Accepted and proposed cryptic couplings in oxic N cycling. a15NH4+tracer is added to oxic sediments to mix with14NH4+in the porewater, with the fraction of15N labelling known asFA. Through reactions 1 and 2,14NH4+and15NH4+are oxidised aerobically to14,15NO2−and14,15NO3−to generate a14,15NOx−pool with15N labelling known asFN. NO3−and/or NO2−can be denitrified to N2gas (reactions 3a, 3b), or NO2−can oxidise NH4+anaerobically through anammox to N2gas (reaction 4). Regardless of the precise setting and combination of reactions, all substrates and products are free to mix and the measured ratio of29N2to30N2produced (R) can be predicted from the measured15N labelling in the porewater. The downwards pointing orange arrow indicates NO3−respiration to NO2−that we do not consider further here.bIn contrast, our measured values forRcannot be predicted using the measured fraction of15N labelling in the porewater (FAandFN) and known combinations of reactions 1 to 4 but can only be approximated assuming a cryptic element (FNcry). A cryptic element could be a hidden substrate pool (6, novel or known) or novel parts of existing processes (7, e.g., complete nitrifier-denitrification beyond N2O to N2) and/or a completely new pathway (reaction 5 e.g., complete aerobic ammonia oxidation to N2) or cryptic combinations of known pathways after partial aerobic ammonia oxidation to nitrite (reactions, 1, 3b, 4). 2.32, 95% CI 2.01 to 2.64 versus 2.43, 95% CI 2.12 to 2.74, see Table 2 and Supplementary Table 2 for 29 N 2 and 30 N 2 production). We then repeated our incubations with just 15 NH 4 + (with and without ATU, Treatments 1 and 2) across twelve rivers and measured a similar value for R of 1.8 (95% CI, 1.41 to 2.20, Fig. 3c ) at an even lower value for F N (see Table 1 ). 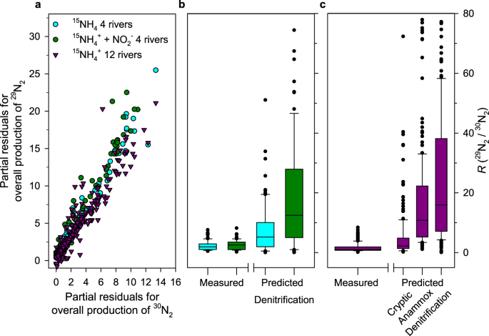Fig. 3: Ratios of29N2and30N2production consistently below those predicted. aConsistent29N2production (nmol g−1h−1) from15N-ammonia added to oxic sediments, against each corresponding measure of30N2production at each time-point (>0.5 h < 10 h) in each incubation in Fig.1apresented here as the partial residuals from mixed-effects models (n= 100 andn= 300, for the 4- and 12-river datasets, respectively).bThe corresponding measured values forRfroma, for the first 4 rivers incubated with either15NH4+(95% CI forR= 2.01 to 2.64) or15NH4+and additional14NO2−(95% CI forR= 2.12 to 2.74), against those predicted for denitrification of porewater NO2−.cMeasuredRvalues for the 12 river sediments incubated with only15NH4+(95% CI forR= 1.41 to 2.20), against predictedRvalues for denitrification, anammox, and a cryptic coupling. See main text and Table2. Upper and lower box boundaries are 75th and 25th percentiles, respectively, upper and lower whiskers are 90th and 10th percentiles, respectively, the extreme outliers the maxima and minima and the horizontal line the centre, median value. 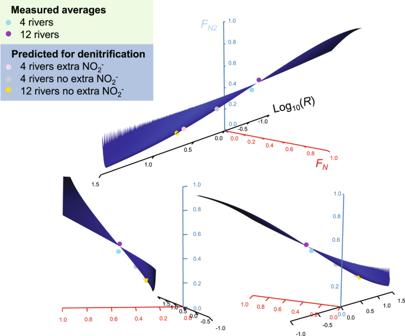Fig. 4: Orientations of the solution space ribbon with both measured and predicted values forR. Here we present all data in just one solution space for the average fraction of15N in the ammonia pool (FA) of 0.51 and combinations of Eq. (8) (FN2) and 9 (ra) both yielding values between > 0 < 1.Ris the ratio of29N2to30N2andFNandFN2the fraction of15N in the NOx−and N2gas pools, respectively. To plotFN2for each of our measured values ofRwe have to assume thatFNequalsFAmeasured in the porewater. In the solution space, there are no solutions whereFA=FN(i.e., 0.51) and this singularity appears as a gap in the ribbon. Despite measurable changes in porewaterFN, the average values for both the 4-river and 12-river study appear near to each other and the gap whereFA=FN. Note that the better parameterised 12-river average touches the gap and by inference,FA≈FNcry(Fig.2b). Denitrification fuelled by porewater NOx−predicts values away from our measured values forR. Note, for the single predicted denitrificationRvalues we use the medianFNvalues. Note, we might have expected R to increase steeply as an inverse function of F N (Supplementary Figure 3 ). We can predict what values for R we might have expected if our N 2 gas had been produced by either denitrification or anammox fuelled by porewater nitrite and/or ammonia, respectively (Fig. 2a ) and compare them to our measured R values to highlight the disparity between the two (Fig. 3b , c and Table 2 ): 
    Predicted R for denitrification,   R = 2 × F_N ×( 1 - F_N)/F_N^2
 (6) 
    Predicted R for anammox,   R = ( 1/F_N - 1) + ( 1/F_A - 1)
 (7) Our measured R values were too low to be explained by either denitrification or anammox fuelled by porewater F N and/or F A (Fig. 2a ) and even a mixture of these two processes couldn’t produce such low values for R on average. This consistent disparity between our measured and predicted values for R , according to the accepted model, along with the constancy in R , despite differences in F N (Table 2 ), strongly implies that porewater NO x − had little influence on the 15 N-labelling of the N 2 gas produced from the oxidation of 15 N-ammonia. Further, in an analogous set of incubations where we added 15 N-nitrite instead of 15 N-ammonia, we measured no consistent production of 15 N-N 2 gas (Treatments 5 & 6 Table 1 and Methods). Hence, nitrogen for N 2 formation was not drawn primarily from the porewater NO x − pool (Fig. 2a ). Instead, we propose that any N 2 producing pathways draw from a cryptic nitrogen pool (Fig. 2b ) with 15 N-labelled fraction, F N cry , instead of the familiar porewater pool with 15 N-labelled fraction, F N pw . Indeed, if we invoke a cryptic pool by making the 15 N-labelling of F N the same as 15 N-ammonia in the porewater F A in Eqs. ( 6 ) and ( 7 ) and thereby force denitrification and/or anammox to draw on that F N cry pool, then the predicted R values come closer to our measured R values ( R cryptic, Fig. 3c and Table 2 ). Fig. 3: Ratios of 29 N 2 and 30 N 2 production consistently below those predicted. a Consistent 29 N 2 production (nmol g −1 h −1 ) from 15 N-ammonia added to oxic sediments, against each corresponding measure of 30 N 2 production at each time-point (>0.5 h < 10 h) in each incubation in Fig. 1a presented here as the partial residuals from mixed-effects models ( n = 100 and n = 300, for the 4- and 12-river datasets, respectively). b The corresponding measured values for R from a , for the first 4 rivers incubated with either 15 NH 4 + (95% CI for R = 2.01 to 2.64) or 15 NH 4 + and additional 14 NO 2 − (95% CI for R = 2.12 to 2.74), against those predicted for denitrification of porewater NO 2 − . c Measured R values for the 12 river sediments incubated with only 15 NH 4 + (95% CI for R = 1.41 to 2.20), against predicted R values for denitrification, anammox, and a cryptic coupling. See main text and Table 2 . Upper and lower box boundaries are 75th and 25th percentiles, respectively, upper and lower whiskers are 90th and 10th percentiles, respectively, the extreme outliers the maxima and minima and the horizontal line the centre, median value. Full size image Table 2 Summary of the overall measured and predicted ratios of 29 N 2 to 30 N 2 production ( R ) for treatments 2 and 4 and the fraction of 15 N labelling in each substrate pool for F N and F A , on average. Overall measured and predicted R estimates, standard errors (s.e.) and 95% confidence intervals were derived with mixed-effects models using lme4 and emmeans (See Methods) and similarly for F N and F A . See Supplementary Table 3 for further details. Full size table N 2 is produced from ammonia through a cryptic intermediate We can use both the accepted [21] and a new mathematical framework to more formally justify our proposal for a cryptic intermediate pool or process. First, we define the proportion of N 2 gas coming from anammox relative to denitrification that is conventionally known as ra [15] . ra has to lie between 0 and 1 and, in the accepted framework, is expressed as a function of porewater F A and F N and R according to [21] (See Eq. (1) to (14) in Supplementary Note 1 ): 
    ra = (R + 2) × F_N^2-2 × F_N/(F_N-F_A) × [(R + 2) × F_N-1]
 (8) In the accepted framework, however, our measured values for R and porewater F A and F N generate nonsensical estimates for ra (e.g., −6.06 to 3.03, not > 0 < 1). Just as for Fig. 3c , we cannot apportion N 2 gas between anammox and denitrification drawing on porewater F N and/or F A – in the conventional sense – to produce our measured R values (Fig. 2a ). Next, we define the 15 N- labelling of the N 2 gas produced ( F N2 ), which, like ra (Eq. 6 ), also has to lie between 0 and 1 (See Eq. (1) to (14) in Supplementary Note 1 ). F_N2 = F_N - R × F_N + 2 × (F_N-1)/2 × (R + 2 - 1/F_N)
 (9) Unlike ra , which is expressed as a function of both porewater F A and F N , only F N is required to parameterise F N2 (Eq. 9 cf . Eq. 8 ). That is not to say that F A has no influence on F N2 , as F N —be it either the F N cry or F N pw pools—must result from ammonia oxidation drawing on F A (Fig. 2 ). We can then use solutions to Eqs. ( 8 ) and ( 9 ) between > 0 < 1 to define a solution space for any combination of F N , F A , and realistic values for R (See Supplementary Figure 3 for R as a function of 15 N atom %) that we can visualise as a 3D ribbon (Fig. 4 ). The height of the ribbon is defined in terms of F N2 and is depicted here for our average value for F A of 0.51 (Table 1 and see Supplementary Fig. 4 for F A at 0.1 and 0.9). Overall the ribbon is very narrow and where F A = F N there are no solutions and this singularity appears as a gap in the ribbon. If F N cry is isolated and derives solely from the oxidation of F A (Fig. 2b ), then F N cry has to equal F A . Further, if F N 2 is only dependent on F N (Eq. 9 ) and this F N is equivalent to F N cry , then our calculated values for F N2 —plotted as functions of our measured values for R and F A (where F N cry equal F A )—should fall near the gap in the ribbon where F N equals F A . This is indeed what we observe and especially for the better parameterised 12 river estimate (Fig. 4 ). In contrast, if we again force denitrification to be the only source of N 2 , and calculate F N2 assuming that F N = F N pw (Fig. 2a ), then the points fall away from our measured R values. Hence, in the presence of 15 N-ammonia and oxygen, our measured R values only make sense if we assume F N cry = F A (Fig. 2b ) i.e., the porewater nitrite pool essentially represents the left-overs of the cryptic transformations during which N 2 is produced. Fig. 4: Orientations of the solution space ribbon with both measured and predicted values for R . Here we present all data in just one solution space for the average fraction of 15 N in the ammonia pool ( F A ) of 0.51 and combinations of Eq. ( 8 ) ( F N 2 ) and 9 ( ra ) both yielding values between > 0 < 1. R is the ratio of 29 N 2 to 30 N 2 and F N and F N 2 the fraction of 15 N in the NO x − and N 2 gas pools, respectively. To plot F N 2 for each of our measured values of R we have to assume that F N equals F A measured in the porewater. In the solution space, there are no solutions where F A = F N (i.e., 0.51) and this singularity appears as a gap in the ribbon. Despite measurable changes in porewater F N , the average values for both the 4-river and 12-river study appear near to each other and the gap where F A = F N . Note that the better parameterised 12-river average touches the gap and by inference, F A ≈ F N cry (Fig. 2b ). Denitrification fuelled by porewater NO x − predicts values away from our measured values for R . Note, for the single predicted denitrification R values we use the median F N values. Full size image Internal NO x − cycling or a novel pathway or organism We propose that the coupling between ammonia oxidation and N 2 gas production in oxic, permeable riverbed sediments involves a cryptic intermediate pool derived solely from the oxidation of ammonia that remains isolated from the porewater prior to the production of N 2 gas. In one scenario, a cryptic pool, similar to the porewater NO x − pool, is fed by the oxidation of ammonia to NO x − , or possibly NO (ref. [3] , [23] , [24] ), through nitrification. The pathway from F N cry to the production of N 2 gas, however, branches off before that NO x − mixes with the ambient porewater NO x − (Fig. 2b ) and would require internal NO x − cycling. Internal NO x − cycling is recognised as a potential source of interference for 15 N isotope tracer studies in the ocean [25] , [26] and is known in the consortia of ammonia oxidisers and anammox bacteria in wastewater CANON [27] reactors (Complete Autotrophic Nitrogen removal Over Nitrite. Figure 2b , reactions 1 & 4) – though the actual mechanism in nature remains unknown. Alternatively, some aerobic ammonia oxidising bacteria first produce nitrite (reaction 1) that they then reduce to N 2 O gas in a process known as nitrifier-denitrification [3] . Known nitrifier-denitrifier bacteria, however, lack a canonical N 2 O-reductase (NOS, nosZ ) to reduce N 2 O to N 2 gas, so are not currently recognised as complete denitrifiers (reaction 7, Fig. 2b ). Nitrosocyanin, a soluble red Cu protein isolated from Nitrosomonas europaea [28] , is recognised as a plausible substitute to canonical N 2 O-reductase that could enable complete nitrifier-denitrification to N 2 gas [3] . Our data enable us to test this hypothesis. For example, we know that 15 NO 2 − from the initial oxidation of 15 NH 4 + exchanges with the porewater (reaction 1, Figs. 1 b and 2a ) and we would expect, therefore, that 15 NO 2 − added to the porewater would be available to any nitrifying-denitrifying bacteria [29] . We have, however, already shown that adding 15 NO 2 − to the porewater resulted in no consistent production of N 2 gas (Treatments 5 & 6, Table 1 ) i.e., N 2 gas production is dependent on the initial oxidation of 15 N-ammonia. This fact, along with the clear discrepancy between the measured and predicted scenarios involving porewater NO x − (Figs. 3 b, 3 c & 4 ) make it hard to reconcile our N 2 gas production with either nitrifier-denitrification or canonical denitrification (reactions 3a, 3b & 7, Fig. 2 ). Finally, it is theoretically possible for ammonia to be completely oxidised by oxygen to N 2 gas (equation 5 [8] ) within a single, unknown organism. Such a reaction offers the simplest explanation for our results, with their strong dependency on aerobic ammonia oxidation and lack of influence from external porewater nitrite. Regardless of the actual pathway that produces the N 2 gas (Fig. 2b ), an isolated cryptic intermediate pool has to have the same 15 N-labelling of the ammonia pool ( F N cry = F A ). As a consequence of this equality, we can no longer distinguish between sources of N 2 gas, be it a denitrification-like pathway reductively combining N from an oxidised cryptic pool, an anammox-like process drawing on ammonia and cryptic N, or complete ammonia oxidation, as they would all produce 29 N 2 and 30 N 2 at the same ratio (Fig. 2b where R is equal for each process). Our observations challenge the current understanding of a key coupling in the nitrogen cycle in permeable, oxic riverbed sediments that may also apply to other biomes where the oxidation of ammonia is tightly coupled to the production of N 2 gas, such as continental shelf-sediments [30] , [31] and groundwater aquifers [17] . Whether it transpires that our cryptic coupling is mediated by a novel organism or, as of yet, a masked combination of known players in the nitrogen cycle remains to be resolved. Study sites and sediment sampling We began by collecting sediment samples from four rivers which we subsequently widened to a total of twelve rivers in southern England, UK, between October 2015 and May 2016 (Supplementary Figure 1 and Supplementary Table 1 ). Among them, the Rivers Lambourn, Darent, Wylye, Rib, Pant, Stour (1) and Stour (2) have chalk-based, permeable gravel-dominated riverbeds, while the Rivers Marden, Hammer, Medway, Broadstone, and Nadder have less permeable, sand-dominated riverbeds as described elsewhere [18] , [32] , [33] . At each river, surface sediments (<5 cm) were collected from five different locations using Perspex corers (13-cm × 9-cm internal diameter, 827 mL and sealed at one end with an oil-seal stopper)) which were then transferred to plastic zip-lock bags (VWR International) and stored in a cool bag (Thermo) during transport back to the laboratory. Each sediment sample from each river was then homogenised in the laboratory for the experiments described below. Aerobic ammonia oxidation in oxic sediment slurries 15 N-NH 4 + oxidation experiments were carried out with sediments first from four rivers (the rivers Lambourn, Wylye, Marden, and Hammer) and then all twelve. In a standard anoxic application of 15 N isotope pairing techniques [34] , [35] , [36] , ambient porewater nitrite, nitrate, and any residual oxygen are removed by pre-incubating the anoxic sediment slurries for 12 h to 24 h before adding any 15 N-tracers [35] , [36] . Here this was not possible as we were measuring the aerobic oxidation of NH 4 + and so to avoid contamination from the high background 14 NO x − ( 14 NO 3 − + 14 NO 2 − ), which is typical for these rivers [24] , instead we used nitrite- and nitrate-free synthetic river water (0.12 g/l NaHCO 3 , 0.04 g/l KHCO 3 , 0.07 g/l MgSO 4 . 7H 2 O, 0.09 g/l CaCl 2 2H 2 O, pH = 7) to make the sediment slurries as before [18] . Oxic slurries were prepared by adding approximately 3 g sediment (~0.75 ml of porewater) and 2.7 ml air-saturated synthetic river water into 12 ml gas-tight vials (Exetainer, Labco), leaving an approximate 6 ml headspace of air which is equivalent to ~58 µmol O 2 per prepared vial. We know from previous incubations with similar sediments from 28 rivers [37] respiration rates to be ~187 nmol O 2 g −1 h −1 , on average (±64.3, 95%, C.I. ), that would consume ~12% of the total oxygen during a 12 h incubation. In addition, we also checked oxygen over time using a microelectrode (50 µm, Unisense) in parallel sets of scaled-up slurries (120 mL with the same ratio of sediment to water to headspace) for two rivers and found comparatively little consumption as before [18] and see example in Supplementary Figure 2 . To trace the oxidation of ammonia to N 2 gas, the prepared oxic slurry vials were then sealed and injected with 100 µl of 14 mM 15 NH 4 + stock-solutions (98 atom% 15 N, Sigma-Aldrich) to generate final porewater concentrations of ~390 µM 15 NH 4 + . This high 15 N concentration ensured sufficient labelling of the ammonia pool (~50%) to enable quantifiable production of both single-labelled, 29 N 2 , and dual-labelled, 30 N 2 , in order to calculate R in Eqs. ( 6 ) to ( 9 ). To link the production of N 2 gas to the initial aerobic oxidation of ammonia, an additional set of slurries were injected with 100 µl of 14 mM 15 NH 4 + (as above), along with 2.8 mM (stock-solution) of the ammonia mono-oxygenase inhibitor [19] , allylthiourea (ATU), to give final porewater concentrations of ~390 µM 15 NH 4 + and ~80 µM ATU. While we have shown previously that 80 µM ATU inhibits aerobic ammonia oxidation in gravel and sandy riverbed sediments [18] , higher concentrations maybe required in other settings [38] . All of the oxic slurry vials were then incubated on a shaker (120 rpm, Stuart SSL1) for up to 12 h (Table 1 , Treatments 1 and 2) in a temperature-controlled room at 12 °C. Incubations amended with just 15 NH 4 + were terminated at 0 h, 0.5 h, 1 h, 3 h, 4.5 h, 6 h, 9 h, and 12 h while those amended with both 15 NH 4 + and ATU were terminated at 0 h, 3 h, 6 h, and 12 h by injecting 100 μl of formaldehyde (38%, w/v) through the vial septa. All vials were then stored upside down prior to quantification of 29 N 2 and 30 N 2 by mass-spectrometry and R is then simply 29 N 2 / 30 N 2 (see below). In addition to measuring the production of 29 N 2 and 30 N 2 gases ( R ), the fraction of 15 N in the inorganic nitrogen porewater pools ( F A for ammonia and F N for NO x − e.g., NO 2 − plus NO 3 − ) needed to be quantified too (see Eqs. 6 to 9 ). To avoid any potential interference from formaldehyde, on the analysis of the inorganic nitrogen species, a parallel set of 15 NH 4 + amended slurries was prepared solely for nutrient analyses. At each time point (as above for N 2 gas analysis), vials were injected with 20 µL of 1.6 M NaOH to preserve nitrite before being frozen at −20 °C [39] . Samples were defrosted and centrifuged at 1200 rpm for 10 min and the collected supernatant analysed (see below). Manipulating the degree of 15 N-labelling in the porewater NO 2 − pool ( F N as F N pw ) In typical anoxic sediment slurry incubations used to quantify N 2 gas production from denitrification and anammox [34] , [35] , the fraction of porewater substrate labelled with 15 N ( F A or F N ) influences the ratio of 29 N 2 to 30 N 2 produced. To characterise the influence of porewater NO 2 − on the coupling between 15 N-NH 4 + oxidation and 15 N-N 2 production in oxic sediment slurries, we manipulated the fraction of porewater NO 2 − labelled with 15 N. Oxic sediment slurries from the first four riverbeds were injected (100 µl) with combinations of stock-solutions of 14 mM 15 NH 4 + and 840 µM 14 NO 2 − or just 14 mM 15 NH 4 + and both with or without 2.8 mM ATU. This generated final porewater concentrations of ~390 µM 15 NH 4 + , ~24 µM 14 NO 2 − or ~80 µM ATU and the prepared vials were then incubated on a shaker as above (see Table 1 , Treatments 3 and 4). As above, oxic slurry vials were sacrificed at different time points for 15 N 2 gas analysis and with a parallel set of 15 NH 4 + or 15 NH 4 + plus NO 2 − amended slurries solely for nutrient analyses. To further test the dependency of N 2 gas production on the initial oxidation of 15 N-ammonia, we also performed a set of analogous incubations with sediments from the first four rivers with 15 NO 2 − (Table 1 , Treatments 5 and 6). Here everything was the same (amount of sediment, with or without ATU, incubation times, oxygen etc.,) except the 15 N-labelling was added with nitrite rather than ammonia (as above) to final concentrations of ~390 µM 14 NH 4 + and ~24 µM 15 NO 2 − (98 atom% 15 N, Sigma-Aldrich). If active, we would have expected N 2 gas production from reactions 3b and 4. Analytical methods Headspaces of the oxic slurry samples were analysed for 15 N-N 2 using a continuous-flow isotope ratio mass spectrometer (Sercon 20–22, UK) as described elsewhere [18] . The mass spectrometer has a sensitivity of 0.1 ‰ 15 N which here translates to approximately 0.1 nmol 15 N-N 2 g −1 dry sediment. To determine porewater F N (NO 2 − or NO x − , below) the concentration of 15 NO 2 − in the 15 NH 4 + treatments was measured, the preserved supernatants were diluted and 3 ml of sample transferred into a new 3 ml gas-tight vial (Exetainer, Labco), the vial capped and a 0.5 ml helium headspace (BOC) added. Samples were injected with 100 μl of sulfamic acid (4 mM in 4 M HCl) and placed on a shaker (120 rpm, Stuart SSL1) overnight to reduce 15 NO 2 − to 15 N-N 2 and the headspaces subsequently analysed for 15 N-N 2 as above [18] , [40] . For 15 NO x − ( 15 NO 2 − plus 15 NO 3 − ) analysis, 0.3 g spongy cadmium and 200 µl of 1 M imidazole, along with 3.5 ml of sample were added to each gas-tight vial (12 ml, Exetainer, Labco) and the vials shaken (120 rpm, Stuart SSL1) for 2.5 h to reduce 15 NO 3 − to 15 NO 2 − and the samples then treated as above to convert 15 NO 2 − to N 2 [18] , [41] . The sensitivity for 15 NO x − was approximately 0.4 nmol 15 N g −1 dry sediment. F N was then calculated for NO 2 − or NO x − as: 
    F_N =  ^15NO_x^ - /( ^15NO_x^ - +  ^14NO_x^ - )
 (10) And similarly for F A : 
    F_A =  ^15NH_4^ + /(  ^15NH_4^ + +  ^14NH_4^ + )
 (11) Where 15 NH 4 + was determined by the increase in concentration, measured by standard indophenol-blue wet-chemistry, above ambient background in controls after the addition of 15 NH 4 + . Sediment particle size was determined by sorting the dried sediments through a series of sieves (Endecotts Ltd, England) from 16 mm, 13.2, 8, 4, 1.4, 0.5, 0.25, 0.125, to 0.0625 mm and then weighing each size fraction. Grain size distributions were calculated and classified on the Wentworth scale as gravel (particles coarser than 2 mm), sand (particles between 0.0625 and 2 mm), mud (silt plus clay material finer than 0.0625 mm) [42] . For sediment organic C and N content, disaggregated samples were oven-dried, acidified by HCl (2 M) to remove inorganic carbonates [43] and re-dried to a constant weight. Then ~50 mg of sediments were transferred to tin-cups, reweighed, and combusted at 1000 °C in an integrated elemental analyser and mass-spectrometer (Sercon, Integra 2, UK). Statistical analysis We used mixed-effects models to estimate overall rates of total 15 N-N 2 gas production during the incubations (Fig. 1a ), treating each of either the first four or subsequent twelve rivers as genuine, independent replicates. Within each river, each of the 5 technical replicates were nested within each respective river and fitted as random effects on the slope and intercept in each case; though it was not always necessary to retain replicate or all the random effects in a model to get the best fit to the data – based on lowest AIC (Akaike Information Criterion). To visualise the consistent production of 29 N 2 to 30 N 2 across the incubations with 15 N-ammonia, we regressed each measure of 29 N 2 on each measure of 30 N 2 , at each time point, in each incubation and display (Fig. 3a ) the partial residuals for the best fitting model [44] . To estimate the overall average measured and predicted ratios of 29 N 2 to 30 N 2 ( R ) we only used the data for the time points >0.5 h < 10 h i.e., when there was measurable (~0.1 nmol N 2 g −1 dry sediment), steady-production of both 15 N labelled gases, divided each measure of 29 N 2 by each respective measure of 30 N 2 at each time point, in each incubation and treated river and replicate as above. For the first 4 rivers, the ratio R was estimated by fitting each time point as a random-effect, but for the larger, 12 river dataset, time was fitted as a fixed-effect and R estimated for the middle time point in the incubations and similarly for F N (for both NO 2 − and NO x − ) and F A . All statistical analyses were performed in R (version 3.6.3, 2020-02-29) under RStudio (version 1.2.5033). Model fitting was carried out in the “lme4” package (version 1.1-21) and parameter (marginal mean) estimates, standard errors, and confidence intervals derived using the “emmeans” package (version 1.4.5) with Kenwood-Roger degrees of freedom and Tukey correction where appropriate.